Auditory cortex of newborn bats is prewired for echolocation Neuronal computation of object distance from echo delay is an essential task that echolocating bats must master for spatial orientation and the capture of prey. In the dorsal auditory cortex of bats, neurons specifically respond to combinations of short frequency-modulated components of emitted call and delayed echo. These delay-tuned neurons are thought to serve in target range calculation. It is unknown whether neuronal correlates of active space perception are established by experience-dependent plasticity or by innate mechanisms. Here we demonstrate that in the first postnatal week, before onset of echolocation and flight, dorsal auditory cortex already contains functional circuits that calculate distance from the temporal separation of a simulated pulse and echo. This innate cortical implementation of a purely computational processing mechanism for sonar ranging should enhance survival of juvenile bats when they first engage in active echolocation behaviour and flight. Echolocation, as an active sensory system, crucially depends on the design of sonar signals that are adapted to specific foraging situations [1] , [2] . Short downward frequency-modulated (FM) sweeps are used as echolocation calls or call components in all bat species known. The FM signal serves two purposes: it provides information about target surface structure based on spectral changes in the echo and it is used as time marker to allow a precise neuronal calculation of target distance from echo delay [1] , [2] , [3] , [4] , [5] . As a neuronal correlate for target distance calculation, neurons in the auditory cortex (AC) of echolocating bats have been described that selectively respond to pairs of FM stimuli that represent pulse and echo [3] , [6] , [7] , [8] , [9] , [10] . These combination-sensitive neurons are maximally facilitated at specific delays between pulse and echo. The present study investigates the postnatal development of echo delay tuning in the AC of two bat species that differ in foraging behaviour, the frugivorous bat Carollia perspicillata (CP, for discussion of nutrition see ref. 10 ) and the insectivorous moustached bat, Pteronotus parnellii (PP). In adult CP and PP, dorsal cortex neurons strongly respond to pairs of FM signals, mimicking sonar pulse and echo (FM P –FM E ). Neurons responding to different echo delays are chronotopically arranged so that a continuous representation of echo delay time is created on the cortical surface [6] , [10] . For PP, it has been demonstrated that delay-tuned neurons are crucial for temporal discrimination behaviour [11] . The extraction of target distance from echo delay is a purely computational feature established in the ascending auditory system of bats, that unlike frequency tuning, does not directly depend on the receptor surface in the inner ear [3] , [7] , [9] . Therefore, we expected that its neuronal implementation would require periods of experience-dependent plasticity during postnatal development. Instead, we found, that delay-sensitive cortical neurons are already functional at birth, long before they are used for echolocation. In this respect, we conclude that part of the bat AC is prewired before its subsequent use during echolocation. Overview The study combined experiments performed in Frankfurt, where a breeding colony of CP was available, and in Havana, where access to hot cave maternity colonies of PP was possible. In adults of both species, delay-tuned cortical neurons are chronotopically arranged: neurons tuned to short echo delays are positioned more rostrally than neurons tuned to longer delays [6] , [10] ( Fig. 1a ). Although CP only uses short FM calls for echolocation, PP uses CF–FM sonar signals where the downward sweeping FM component is preceded by a long constant frequency (CF) component (see insets in Fig. 1 ). The long CF component does not seem to have a role for target distance calculation, but is an optimal signal for target detection and for analysis of insect wing beat [4] . 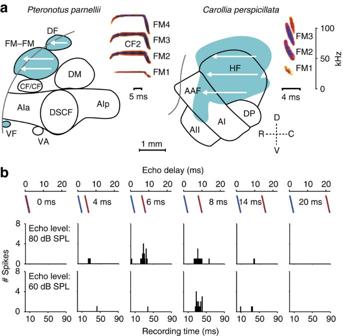Figure 1: Echo delay sensitive areas in bat auditory cortex. (a) Cortex organization in adultP. parnellii(adapted from refs4,38,39, based on physiological and anatomical data) and in adultC. perspicillata(adapted from refs10,37, based on physiological data). Auditory cortex in PP (left) with three delay-sensitive areas FM–FM, DF (dorsal fringe), VF (ventral fringe). Arrows give direction of decreasing characteristic echo delay. DM (dorsomedial area), AIp (posterior AI), AIa (anterior AI), DSCF (Doppler shift constant frequency area), VA (ventroanterior area), DP (dorsoposterior area). Inset: representative spectrogram of echolocation calls with constant-frequency (CF) and frequency-modulated (FM) components. In adult CP (right) delay-sensitive neurons are located in the high-frequency (HF) area and in the border region between the anterior auditory field (AAF), primary auditory cortex (AI) and AII (secondary auditory cortex). (b) Example of neuronal responses to FM call–echo pairs in a 7-day-old CP. Upper row: scheme of presented stimuli with increasing delay between a FM2call and FM2echo component. Middle, lower row: post stimulus time histograms of spike activity of a single neuron during presentation of a FM2call component (level: 90 dB SPL) followed by a FM2echo component. The neuron is tuned to echo delays of 6–8 ms. SPL: sound pressure level, expressed in dB re 20 μPascal. Figure 1: Echo delay sensitive areas in bat auditory cortex. ( a ) Cortex organization in adult P. parnellii (adapted from refs 4 , 38 , 39 , based on physiological and anatomical data) and in adult C. perspicillata (adapted from refs 10 , 37 , based on physiological data). Auditory cortex in PP (left) with three delay-sensitive areas FM–FM, DF (dorsal fringe), VF (ventral fringe). Arrows give direction of decreasing characteristic echo delay. DM (dorsomedial area), AIp (posterior AI), AIa (anterior AI), DSCF (Doppler shift constant frequency area), VA (ventroanterior area), DP (dorsoposterior area). Inset: representative spectrogram of echolocation calls with constant-frequency (CF) and frequency-modulated (FM) components. In adult CP (right) delay-sensitive neurons are located in the high-frequency (HF) area and in the border region between the anterior auditory field (AAF), primary auditory cortex (AI) and AII (secondary auditory cortex). ( b ) Example of neuronal responses to FM call–echo pairs in a 7-day-old CP. Upper row: scheme of presented stimuli with increasing delay between a FM 2 call and FM 2 echo component. Middle, lower row: post stimulus time histograms of spike activity of a single neuron during presentation of a FM 2 call component (level: 90 dB SPL) followed by a FM 2 echo component. The neuron is tuned to echo delays of 6–8 ms. SPL: sound pressure level, expressed in dB re 20 μPascal. Full size image Using stimulation with pairs of FM stimuli mimicking pulse (FM P ) and echo (FM E ), neuronal responses to randomly presented echo levels and delays were sampled while keeping the pulse at a fixed level ( Fig. 1b ) and delay response areas (DRAs) with a characteristic delay (CD) were constructed ( Fig. 2 ). In the case of CP, where neurons best respond to homoharmonic pulse–echo pairs [10] , [12] , FM P –FM E pairs of the same harmonic (for example, FM 2 –FM 2 ) were used as stimuli. In PP, heteroharmonic combinations of a first harmonic FM P and a higher harmonic FM E were applied (FM 1 –FM 2–4 ) [6] . 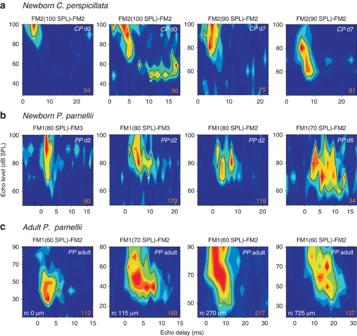Figure 2: Delay response areas (DRAs) of example neurons. Contour plots of response strength are plotted as function of echo delay and echo level. Values for maximum activity (dark red contours) are indicated in spikes per second by orange numbers at the bottom right. Dashed line indicates 50% of maximum activity, white asterisks indicate curve minimum (characteristic delay). Top right: animal age. The call–echo combination is indicated above each plot. (a) Newborn CP: DRAs tuned to 3–12 ms recorded between postnatal days 0–7. (b) Newborn PP: DRAs tuned to 2–10 ms from postnatal days 2–6. (c) For comparison, DRAs from an adult PP are shown; rostro-caudal position is given in μm at the bottom left. In newborn bats, the shape of DRAs is comparable to those of adults although the levels of both call and echo required to obtain responses are higher than in adults. Figure 2: Delay response areas (DRAs) of example neurons. Contour plots of response strength are plotted as function of echo delay and echo level. Values for maximum activity (dark red contours) are indicated in spikes per second by orange numbers at the bottom right. Dashed line indicates 50% of maximum activity, white asterisks indicate curve minimum (characteristic delay). Top right: animal age. The call–echo combination is indicated above each plot. ( a ) Newborn CP: DRAs tuned to 3–12 ms recorded between postnatal days 0–7. ( b ) Newborn PP: DRAs tuned to 2–10 ms from postnatal days 2–6. ( c ) For comparison, DRAs from an adult PP are shown; rostro-caudal position is given in μm at the bottom left. In newborn bats, the shape of DRAs is comparable to those of adults although the levels of both call and echo required to obtain responses are higher than in adults. Full size image Cortical delay tuning in neonates Delay-tuned neurons could already be characterized in the earliest developmental stages (CP: day 0; PP: day 1) at cortical positions that correspond to the adult FM–FM area in PP or to the high-frequency (HF) fields in CP ( Fig. 2 ). Neonatal bats from the two species do not actively fly or echolocate within a period extending to at least 8 days after birth [13] , [14] . In the case of PP, the neonatal bats hang at fixed locations in their maternity caves, are rather immobile and wait for their mothers to return from hunting. CP neonates are carried by their mothers during flight. To evoke delay-tuned responses in newborn bats, stimuli at higher levels than in adults had to be used, possibly to compensate for reduced sensitivity of the immature peripheral auditory system [15] . Both in bats studied between postnatal day 0–7 animals and in adults, neuronal DRAs tuned to longer echo delays are often tilted such that the preferred echo delay decreases with increasing echo level (examples in Fig. 2 , Supplementary Fig. S1 ; see also ref. 12 ). Chronotopy within the first postnatal week In neonates where we could sample a sufficient number of neurons at different rostro-caudal positions, a clustering of units tuned to short versus long echo delays became apparent. In a 3-day-old PP, neurons tuned to delays of 1–5 ms are located at more rostral positions than units tuned to longer delays of 10–21 ms ( Fig. 3a ). In data collected from this individual, the response area of neurons sensitive to long echo delay was much larger than that of the short delay units. When using the extension of the adult FM–FM region as reference (outlines in Fig. 3a ), the delay-tuned area was located at the ventro-rostral part of the FM–FM area, close to a dominant sulcus. In the neonates, cortical regions that would correspond to the caudal FM–FM area in adults were not responsive to pure tones or FM–FM pairs. As in the adult ventral FM–FM region [3] , the neurons responded best to stimulus pairs containing a second harmonic FM E . In CP, developmental changes of chronotopy could be studied by pooling data from a number of animals that were of the same age within±1 day ( Fig. 3b ). In adults, data pooling has been shown to yield a map quality similar to that of individual maps [10] . For the youngest age group (day 0), only 18 delay-tuned neurons could be mapped primarily in the centre region of the HF area. Although the chronotopic gradient is slightly below significance ( P =0.12; Wilcoxon ranked sum test), the preferred direction of increasing echo delay representation is already at an angle that is comparable to that in older bats. In the 0-day-old bats, as well as in the older animals, units that were not responsive to FM pairs but did react to pure tones were recorded in primary auditory cortex (AI), anterior auditory field (AAF), HF and dorsoposterior area. For bats of day 7–28, the chronotopic gradient was highly significant, covered the whole HF area and reached ventrally into the HF border region between AI and AAF, similar to adults. 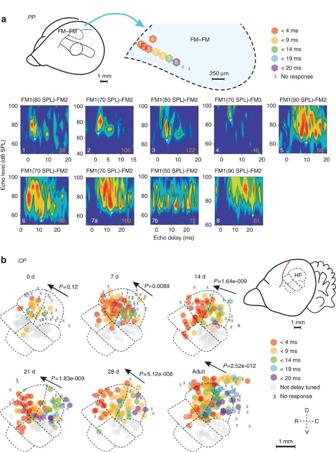Figure 3: Development of chronotopy. (a) DRAs recorded in a 3-day-old PP. Top scheme: positions of penetrations in relation to adult FM–FM area. The penetrations are numbered from 1 to 8 and corresponding DRAs are shown below with the penetration number (in white) given at bottom left. The maximum number of spikes is given at bottom right (in orange). DRAs are arranged in a rostral cluster of units responding to short delays and a caudal region with units tuned to long delays. DRA tuning width increases at longer delays. For unit 7, responses at a call level of 50 dB SPL (7b) are not delay-specific, the unit responds to echo levels of about 65–80 dB SPL. Increasing the call level to 70 dB SPL (7a) induces inhibition for up to about 5 ms echo delay, followed by delayed facilitation, which together produces a well-defined DRA. (b) Position of units with different CD (colour coded) in CP of different age. The data are pooled from 5 bats (day 0, day 7), 6 bats (day 14), 4 bats (day 21), 3 bats (day 28) and 13 bats (adult). The arrows indicate optimal direction of chronotopy towards short CDs; theP-values give the correlation probability. Figure 3: Development of chronotopy. ( a ) DRAs recorded in a 3-day-old PP. Top scheme: positions of penetrations in relation to adult FM–FM area. The penetrations are numbered from 1 to 8 and corresponding DRAs are shown below with the penetration number (in white) given at bottom left. The maximum number of spikes is given at bottom right (in orange). DRAs are arranged in a rostral cluster of units responding to short delays and a caudal region with units tuned to long delays. DRA tuning width increases at longer delays. For unit 7, responses at a call level of 50 dB SPL (7b) are not delay-specific, the unit responds to echo levels of about 65–80 dB SPL. Increasing the call level to 70 dB SPL (7a) induces inhibition for up to about 5 ms echo delay, followed by delayed facilitation, which together produces a well-defined DRA. ( b ) Position of units with different CD (colour coded) in CP of different age. The data are pooled from 5 bats (day 0, day 7), 6 bats (day 14), 4 bats (day 21), 3 bats (day 28) and 13 bats (adult). The arrows indicate optimal direction of chronotopy towards short CDs; the P -values give the correlation probability. Full size image Postnatal maturation of characteristics of time sensitive neurons To assess distribution, sensitivity and tuning width of DRAs at different stages, a comparison was made among neonates in the first postnatal week (days 0–7) that did not yet echolocate, bats of intermediate age (days 20–28) that did echolocate and were capable of flight, and adults. In all three age groups and in both species, the distribution of CDs was comparable with an overrepresentation of units coding delays between 2 and 8 ms ( Supplementary Fig. S2 ). The sensitivity at CD increased with increasing age ( Fig. 4a ). For PP, day 0–7 animals had average CD thresholds of 70±11 dB SPL (sound pressure level, expressed in dB re 20 μPascal) with the youngest animals (days 0–2, red circles in Fig. 4a ) slightly less sensitive (79±11 dB SPL). Threshold decreased to 56±13 dB SPL in day 20–28 animals and reached 50±14 dB SPL in adults. For all age groups, CP was 2–6 dB more sensitive than PP (days 0–7: 64±15 dB SPL; days 20–28: 54±12 dB SPL; adult: 44±9 dB SPL). The data for anaesthetized adult PP are comparable to published data on awake bats [3] , [6] , [7] , [16] , [17] . The threshold decrease of neurons that were grouped into short, medium and long CD units ( Fig. 4b ) was largest and most significant between day 0–7 and day 20–28 animals for all delays in PP and for short and medium delays in CP. Thresholds for long delays decreased significantly only between day 0–7 animals and adults in CP. The tuning width of DRAs, measured 10 dB above CD, was rather stable over all age groups ( Fig. 4b ). In the youngest bats ( Fig. 2 ) sharply tuned neurons were already present. The only significant decrease of tuning width with age was found for PP short CD neurons. In CP, there was no significant change of tuning width between day 0–7 animals and adults, and the tuning width of short CD neurons increased between day 20–28 animals and adults. In both bat species, the latency of delay-tuned responses, measured from PSTH histograms, in general increased with increasing echo delay. However, the response latencies of different neurons tuned to the same echo delay range varied considerably in all age groups ( Supplementary Fig. S3 ) and developmental changes were not obvious. 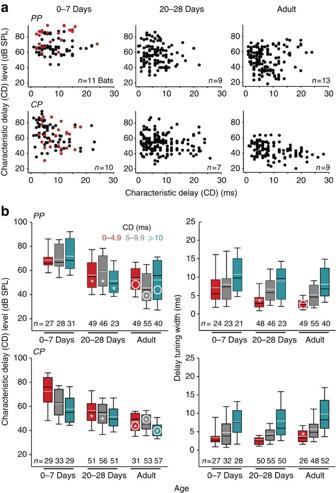Figure 4: Age-dependent changes of delay tuning. (a) CD and echo threshold levels at CD for three age groups (0–7 days, 20–28 days, adult) for both species. Red symbols: youngest animals, days 0–2. (b) Comparison of CD threshold level (left) and DRA-tuning width (right) for the three age groups. CD threshold significantly decreases with increasing age (P<0.01; Wilcoxon ranked sum test; asterisks indicate significance compared with the next younger age group, circles indicate significance between the 0–7 days and adult group). Neurons are sorted into three CD groups (0–4.9, 5–9.9 ms, ≥10 ms, see inset). Number of neurons for each box plot is given below the plot. In PP, the tuning width of neurons tuned to 0–4.9 ms significantly decreases between the youngest and the intermediate and adult age group. Box plots delimit 50 and 75% with geometric (white line) and arithmetic (black line) mean. Figure 4: Age-dependent changes of delay tuning. ( a ) CD and echo threshold levels at CD for three age groups (0–7 days, 20–28 days, adult) for both species. Red symbols: youngest animals, days 0–2. ( b ) Comparison of CD threshold level (left) and DRA-tuning width (right) for the three age groups. CD threshold significantly decreases with increasing age ( P <0.01; Wilcoxon ranked sum test; asterisks indicate significance compared with the next younger age group, circles indicate significance between the 0–7 days and adult group). Neurons are sorted into three CD groups (0–4.9, 5–9.9 ms, ≥10 ms, see inset). Number of neurons for each box plot is given below the plot. In PP, the tuning width of neurons tuned to 0–4.9 ms significantly decreases between the youngest and the intermediate and adult age group. Box plots delimit 50 and 75% with geometric (white line) and arithmetic (black line) mean. Full size image The significant finding of our study is that basic features of cortical representation of external space in the form of echo-delay-tuned neurons are already established before bats actively explore their surroundings by echolocation. This was unexpected, as in contrast to frequency tuning, which is largely inherited from the cochlea, neuronal delay processing is a purely computational feature that is not established before the midbrain level in bats [18] , [19] . We would have expected a progressive development of delay-tuned cortical responses in parallel to the behavioural use of echolocation. Specifically, we expected that young bats that are not yet able to actively echolocate up to their second postnatal week [13] , [14] would either lack combination-sensitive delay-tuned responses or exhibit broad tuning to echo delay. It is conspicuous that at the same developmental stage when delay-sensitive neurons are already functional, frequency tuning in the ventrally located primary AC is still quite immature because of ongoing inner ear development. In addition, other forms of facilitative combination sensitivity, reported for adult primary AC are still absent during the first postnatal week [20] . Therefore, one of the neuronal characteristics most crucial and advanced in terms of echolocation processing seems to appear first and not last in the maturation hierarchy of AC. Our results from neonatal bats of two species adapted to different feeding and echolocation strategies emphasize that certain forms of neuronal circuitry for spatial orientation are implemented before their first use as it has also been suggested for hippocampal place units in rodents [21] , [22] . In bats, hippocampal place cells resemble those in rats quite well [23] , [24] and cortical delay-tuned neurons may constitute one of several input features for spatial representation and memory in hippocampus. For this study, we chose two bat species with prominent cortical DRAs and a chronotopically arranged delay-tuned cortical substrate. Chronotopy could enable a rather simple readout of target distance information for behavioural purposes. However, a chronotopic gradient is not a cortical feature absolutely necessary for successful target-range calculation, as dorsal AC of bat species like Eptesicus fuscus and Myotis lucifugus is not chronotopically organized (reviewed in ref. 25 ) and mechanisms relying on population coding, accumulative response integration and periodicity pitch can contribute to target-range perception [9] , [26] , [27] . In particular, the extraction of periodicity pitch that, similar to delay tuning, would involve neuronal delay lines and/or oscillations could be a general principle for analysis of communication sounds in a variety of vertebrates and also very useful for echolocation with its highly repetitive signal sequences [27] . In this respect, it is noteworthy that in PP the delay-tuned dorsal cortex neurons also respond strongly to communication signals [28] . Our data demonstrate that there is an innate selectivity for echo delay. This parallels behavioural evidence that human infants are innately capable of discriminating the timing relations between phoneme pairs [29] . Of course, this does not rule out plasticity and experience-dependent changes in delay tuning during maturation, as it has been demonstrated for other auditory-processing features in mammals (for example, see refs 30 , 31 , 32 ). As we did not manipulate the bats' vocalizations, we cannot exclude that experience-dependent circuits may be refined later on by feedback from the bat's own vocalizations as it has been shown for side-band inhibition and FM-direction sensitivity in postnatal development of the pallid bat's AC [33] , [34] . There is also the possibility that anaesthesia masked some of the possible changes in the maturation of inhibitory circuits, although data on adult awake and anaesthetized PP are comparable in terms of sensitivity and sharpness of delay tuning [3] , [12] . As long-term plasticity in echo delay tuning has been demonstrated in adult PP [35] , a corresponding fine tuning of delay sensitivity should be expected in subadults as it could appear in the form of small developmental changes in tuning width and shape of part of the DRAs ( Fig. 4b , Supplementary Fig. S1 ). The age-related increase in sensitivity of involved cortical delay-tuned neurons, however, is most likely not dependent on experience but produced by maturation of the cochlea (PP: ref. 15 ) as it has been suggested for development of the primary AC of PP [20] . In the ascending auditory system, delay-sensitive neuronal responses are first created at the midbrain level (PP: refs 18 , 19 ). This implies that corresponding collicular circuits should be established already in newborn bats and this may be one reason why cortical delay tuning is functional within the first days of life. An innate implementation of certain features of echolocation has also been demonstrated in young Myotis emarginatus bats that interpreted smooth metal surfaces as water surfaces and approached them to drink without prior experience [36] . So it seems that important components of active orientation systems are neuronally established a priori in a way that allows a certain degree of successful interaction with their surroundings. Animals and experimental conditions For electrophysiological recordings in CP, 24 young bats and 9 adults from our breeding colony in Frankfurt were used. Pregnant females were monitored shortly before giving birth, which enabled us to record in young bats within 24 h after birth (day 0) and at days 7, 14, 21, 28 and 35. PP cannot be bred in sufficient numbers in captivity and were caught in Cuban caves, experiments in 33 young bats and 13 adults took place at Havana University. Age was determined from forearm length [14] , [15] , [20] . Newborns have a forearm length of ~20 mm and the growth rate is ~1 mm per day. For species comparisons at similar age stages, we defined age groups of 0–7 days (CP: 0 and 7 days old, n =10; PP: 1–7 days, n =11) and 20–28 days (CP: 20 and 28 days old, n =7; PP: 20–27 days, n =9). In some of the young bats, we recorded echolocation calls and verified that in PP spontaneous calls first appeared not before day 9 (ref. 14 ) and in CP not before day 17 (ref. 13 ). Individuals of the 0–7 days group did not actively fly or echolocate. At this age, they are carried by mothers (CP) or hang rather immobile in maternity colonies while their mothers are hunting (PP). Bats of the 20–28 days group could fly and were echolocating. Surgical procedure Regarding anaesthesia, the two species are not fully compatible and young bats generally were more susceptible to the anaesthetic. Adult CP were initially anaesthetized with ketamine (10 mg kg −1 Ketavet) and xylazine (38 mg kg −1 Rompun), adult PP with 10 mg kg −1 ketamine and 10 mg kg −1 pentobarbital (Sigma). Young bats <20 days were anaesthetized with ketamine only (CP: 10–20 mg kg −1 , PP: 5–25 mg kg −1 ). Anaesthesia was maintained by regular, usually hourly injection of half the initial dose. A metal bar glued to the skull fixed the animal's head. Craniotomy was performed to expose small areas of the left AC. The location of auditory areas was determined from major blood vessels and, in the case of PP, from the Sylvian fissure and from published cortex maps on adults [3] , [4] , [37] , [38] , [39] and young bats [20] . After experiments, the animals were killed by Pentobarbital overdose and heads were preserved in 4% paraformaldehyde. All experiments comply with the Principles of Animal Care, Publication No. 86-23, revised 1985, of the National Institute of Health, and with the Declaration of Helsinki Principles. The experiments comply with our institute's regulations and were approved by an animal experimentation licence issued by the responsible federal agency (Veterinärdezernat, Regierungspräsidium Darmstadt). Location of recording sites was determined in relation to cortical blood vessels and the Sylvian fissure. For reconstruction of recording sites, photographs of the electrode tips at the recording sites in relation to the skull opening and the blood vessels were made and latter aligned to the fixed brain. In the case of CP, where we had several animals of exactly the same age (±1 day), the individual maps were aligned to composite maps of the respective developmental stage. Recording procedures and data analysis Carbon electrodes (Carbostar-1, Kation Scientific) introduced orthogonally to cortical surface were used to record action potentials extracellularly from single- and multiunits. Most units were recorded at 200–500 μm depth (layers III and IV). The electrode signal was amplified (EX1, Dagan Corp), bandpass filtered (0.3–5 kHz) and was fed into an AD input of a DAP 5200a board (Microstar Laboratories). Downward frequency-modulated FM stimuli (2–5 ms duration, 0.5 ms rise/fall time, 0.4 octaves bandwidth) were generated by DA converters of the DAP board (sampling rate: 385 kHz). Centre frequencies of the FM sweeps were adjusted according to the characteristics of the FM echolocation signals of the respective age group [13] , [14] . For bats of the 0–7 day's group that did not echolocate, the FM centre frequencies were adjusted to multiples of 21–23 kHz (PP) or 30 kHz (CP). A calibrated loudspeaker (ScanSpeak Revelator R2904/7000 or Microtec Gefell MK102.1) was positioned contra-laterally in the right auditory hemifield (about 45° from the midline). The speaker calibration curve, obtained beforehand at a position that corresponded to the bats right pinna, was used to adjust sound levels of pure tones. For the FM stimuli, the centre frequency of the sweep was used for sound level adjustment. For measuring DRAs, FM sweeps mimicking components of the call (FM P ) and delayed echo (FM E ) were presented (repetition period: 250 ms; 4–10 averages). FM P had a constant level within a range of 50–100 dB SPL, FM E was varied randomly in delay and level. To sort action potentials, the first three principle components of spike waveforms were calculated [40] . To separate spikes originating from different neurons, an automatic clustering algorithm 'KlustaKwik' based on the expectation–maximization algorithm was fed with the first three principle components of each spike and then clusters were selected manually [40] . We did not distinguish between single- and multi-unit responses. The responses are treated as multiunits. DRAs were calculated with 50% of maximum response as criterion. The lowest echo level producing this response and the corresponding echo delay (CD) were determined. Neuronal activity was measured within a time window that was adjusted individually to cover all responses to different call–echo combinations. The temporal tuning width of delay tuning curves was measured at 5 and 10 dB above CD level and the maximum of both values was used as tuning width in reference to CD. To assess changes in DRA shape, tilt of the DRA was measured (ms/dB echo level) from linear regression of the echo delay that produces maximum response at different echo levels. In some units the tested echo delay and echo level range were smaller than the full extension of the DRA. Therefore, the number of units usable for tuning width or tilt analysis was smaller than the total number of units (PP: total unit number/tuning width units/tilt units: 348/329/307; CP: 390/367/374). For statistical comparisons, the Wilcoxon ranked sum test was used, with P <0.01 as significance standard. How to cite this article: Kössl, M., Voss, C. et al . Auditory cortex of newborn bats is prewired for echolocation. Nat. Commun. 3:773 doi: 10.1038/ncomms1782 (2012).